A gradient of Bmp7 specifies the tonotopic axis in the developing inner ear The auditory systems of animals that perceive sounds in air are organized to separate sound stimuli into their component frequencies. Individual tones then stimulate mechanosensory hair cells located at different positions on an elongated frequency (tonotopic) axis. During development, immature hair cells located along the axis must determine their tonotopic position in order to generate frequency-specific characteristics. Expression profiling along the developing tonotopic axis of the chick basilar papilla (BP) identified a gradient of Bmp7 . Disruption of that gradient in vitro or in ovo induces changes in hair cell morphologies consistent with a loss of tonotopic organization and the formation of an organ with uniform frequency characteristics. Further, the effects of Bmp7 in determination of positional identity are shown to be mediated through activation of the Mapk, Tak1. These results indicate that graded, Bmp7-dependent, activation of Tak1 signalling controls the determination of frequency-specific hair cell characteristics along the tonotopic axis. Tonotopy, the fundamental organizing principal of the auditory system, refers to the spatial separation and perception of complex sounds based on their component frequencies. Tonotopic organization is present at all levels of the auditory system from the periphery through the brainstem to the cortex [1] . In vertebrates with elongated auditory organs (mammals, birds and some orders of reptiles) tonotopy manifests as a gradient in frequency sensitivity in which hair cells located closest to the saccular end are stimulated by high-frequency sounds while those located at progressively more distal positions respond to lower frequencies. In the chicken auditory organ, the basilar papilla (BP), tonotopic gradients of cell morphology and physiology are present along the proximal-to-distal (tonotopic) axis from as early as E12 (refs 2 , 3 , 4 , 5 , 6 , 7 ). Hair cell density is lowest at the end of the BP located closest to the sacculus (proximal region) and increases progressively in more distal regions ( Fig. 1a–c ). The lumenal surface area of each hair cell also varies along the axis with smaller surface areas present on hair cells located more distally ( Fig. 1a–c ). Similarly, the number of individual stereocilia per hair cell bundle decreases along the tonotopic axis, while the average length of stereocilia per bundle increases [2] , [8] . At the molecular level, numerous proteins are expressed differentially along the BP such as the calcium-binding protein Calbindin, which is more strongly expressed in proximal hair cells but decreases progressively in more distal hair cells [5] , [9] ( Fig. 1a,b ). Furthermore, hair cell physiology also changes along the tonotopic axis, with a gradient in the response kinetics of membrane voltage oscillations forming the basis for frequency-specific electrical tuning [6] , [7] , [10] , [11] , [12] . Tonotopic changes in response kinetics are achieved through interactions between voltage-gated calcium (CaV 1.3 ) channels and large conductance Ca 2+ -activated K + (BK) channels [10] . The β-subunit (Kcnmb1) of the BK channel, which mediates slower response kinetics, is expressed at higher levels in distal, low-frequency hair cells [13] . In addition, as a result of alternative splicing of the nascent pre-mRNA encoding the pore forming α-subunit, graded variations in the structure and kinetics of the BK channel are present along the tonotopic axis of the BP [7] , [10] , [11] , [14] , [15] . 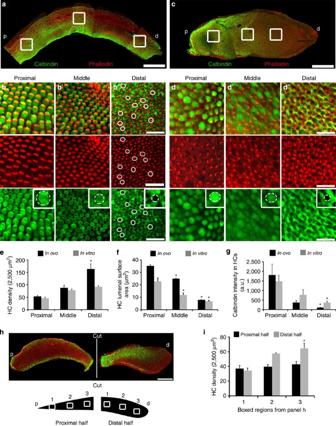Figure 1: Tonotopic organization in the chick basilar papilla develops normallyin vitro. (a) Maximumzprojection of an E12 BP labelled with anti-Calbindin (green) and phalloidin (red) illustrating frequency-specific differences in cell morphology along the tonotopic axis. Proximal (p) and distal (d) ends are indicated. White boxes indicate regions used for zoomed images illustrated inb,b′and b′′. Top panel shows merged calbindin and phalloidin channels. White circles highlight representative hair cells. Middle panel shows phalloidin-labelled stereocilia bundles highlighting the tonotopic differences in hair cell size and number. Lower panels show calbindin fluorescence in hair cells at the same BP regions. Note limited or no expression of Calbindin in hair cells (white circles) inb′′. Insets: high-magnification views of individual hair cell surfaces. (c) Maximumzprojection of a control BP explant, labelled as ina, established at E6.5 and maintained for 6 DIV. As forb–b′′, panels illustrate changes in stereocilia size and density and Calbindin expression along the tonotopic axis. (e–g) Mean hair cell density, lumenal surface area and Calbindin intensity in hair cells in the indicated regions of the BP for samples maintained in ovo (black) orin vitro(grey). In all cases, a gradient is present along the tonotopic axis bothin ovoandin vitro. Fore–g, data are mean±s.e.m. Stars indicate aPvalue<0.05 relative to the proximal value within the same group, based on Student’st-test. (h) Tonotopy is specified before E7.0. Calbindin (green) and phalloidin (red) labelling in proximal (p) and distal (d) halves from an E6.5 BP that was separated at the time of dissection and maintained for 6 DIV. The proximal-to-distal gradient of Calbindin expression is present in the distal half. In contrast, Calbindin expression is almost completely absent in the proximal explant. (i) Quantification of hair cell density from specific regions (see cartoon inh) along proximal and distal explants halves. A gradient of hair cell density is present in distal explants but no change in density is present in proximal explants. Data are mean±s.e.m. Star indicates aPvalue <0.05 relative to box 1, Student’st-test. Fore,n=9 for both conditions, forf,n=8 for both conditions, forg,n=80 cells for each position measured from 4 separate experiments. Scale bars, 100 μm. Figure 1: Tonotopic organization in the chick basilar papilla develops normally in vitro . ( a ) Maximum z projection of an E12 BP labelled with anti-Calbindin (green) and phalloidin (red) illustrating frequency-specific differences in cell morphology along the tonotopic axis. Proximal (p) and distal (d) ends are indicated. White boxes indicate regions used for zoomed images illustrated in b , b ′ and b ′′. Top panel shows merged calbindin and phalloidin channels. White circles highlight representative hair cells. Middle panel shows phalloidin-labelled stereocilia bundles highlighting the tonotopic differences in hair cell size and number. Lower panels show calbindin fluorescence in hair cells at the same BP regions. Note limited or no expression of Calbindin in hair cells (white circles) in b ′′. Insets: high-magnification views of individual hair cell surfaces. ( c ) Maximum z projection of a control BP explant, labelled as in a , established at E6.5 and maintained for 6 DIV. As for b – b ′′, panels illustrate changes in stereocilia size and density and Calbindin expression along the tonotopic axis. ( e – g ) Mean hair cell density, lumenal surface area and Calbindin intensity in hair cells in the indicated regions of the BP for samples maintained in ovo (black) or in vitro (grey). In all cases, a gradient is present along the tonotopic axis both in ovo and in vitro . For e – g , data are mean±s.e.m. Stars indicate a P value<0.05 relative to the proximal value within the same group, based on Student’s t -test. ( h ) Tonotopy is specified before E7.0. Calbindin (green) and phalloidin (red) labelling in proximal (p) and distal (d) halves from an E6.5 BP that was separated at the time of dissection and maintained for 6 DIV. The proximal-to-distal gradient of Calbindin expression is present in the distal half. In contrast, Calbindin expression is almost completely absent in the proximal explant. ( i ) Quantification of hair cell density from specific regions (see cartoon in h ) along proximal and distal explants halves. A gradient of hair cell density is present in distal explants but no change in density is present in proximal explants. Data are mean±s.e.m. Star indicates a P value <0.05 relative to box 1, Student’s t -test. For e , n =9 for both conditions, for f , n =8 for both conditions, for g , n =80 cells for each position measured from 4 separate experiments. Scale bars, 100 μm. Full size image Previous developmental studies have demonstrated that the majority of tonotopic gradients are evident in the BP by E12, suggesting that the signals specifying positional identity must be present before this time. Furthermore, transplantation and in vitro studies demonstrated the development of normal tonotopic identity in BPs isolated as early as E8 refs 16 , 17 ). These results suggest that positional signals are intrinsic to the BP by early embryonic time points but the identity and nature of those signals have not been determined. Given that positional signals are intrinsic to the BP by early time points, we sought to identify and characterize the pathways that establish the tonotopic axis during development. Results of expression profiling identified a gradient of Bone morphogenetic protein 7 ( Bmp7 ) within the developing chick BP at the time of hair cell formation. Modulation of this gradient results in predictable changes in hair cell morphologies that are consistent with different concentrations of Bmp7 inducing specific hair cell phenotypes. These results are consistent with the hypothesis that a gradient of Bmp7 acts to specify positional identity and, therefore, hair cell phenotype along the tonotopic axis of the chick BP. Tonotopic identity in the BP is established before E7 Previous results demonstrated correct development of tonotopy in BPs isolated and maintained in vitro from as early as E8 (refs 16 , 17 ). To determine when the signalling mechanisms specifying tonotopic cues become intrinsic to the BP sensory epithelium, explants were dissected and established in culture from chick embryos between E8 and E6, the youngest age at which such explants would survive. To confirm that tonotopic cues are intrinsic within the BP at early time points, we assayed gradients in cell size and morphology, as well as Calbindin staining, as indicators of establishment of tonotopy ( Fig. 1c,d ). In a normal BP, hair cells are larger and more sparsely populated in the proximal, compared with the distal, region and Calbindin is expressed more highly in proximal hair cells with a progressive decrease towards the distal tip [5] . Results indicate development of tonotopic gradients in hair cell density, hair cell lumenal surface area and expression of Calbindin in hair cells in explants started as early as E6 and maintained for 6 days in vitro (DIV; Fig. 1c–g ). However, outgrowth of stromal cells located at the extreme distal end of BP explants produce some epithelial traction leading to significantly decreased hair cell density in this region. As a result, the most distal end of BP explants was not analysed ( Fig. 1c ). Also, it is important to note that Calbindin is expressed strongly in distal supporting cells, which accounts for the persistence of anti-Calbindin fluorescence in distal regions ( Fig. 1b,d ). Therefore, Calbindin intensity measurements were restricted to the lumenal surfaces of hair cells. While the nature of the cues that specify positional identity are unknown, one hypothesis would be that graded activity of a morphogen could provide instructive cues along the length of the BP [18] . If this model is correct, then hair cell progenitors along the length of the BP would determine their positional identity by interpreting the relative concentration of the morphogen at a particular position along the axis. This would suggest, as is the case for the developing limb bud, that potential sources or signalling centres would reside at either the proximal or distal end of the BP [19] , [20] . To test this hypothesis, we conducted a series of separation experiments in which the BP was dissected and then divided into proximal and distal halves on specific gestational days or half days between E6 and E8. Following separation, proximal and distal halves were established as separate explants and maintained in vitro for 6 days. Separation of the BP at E7 or later results in the development of tonotopically appropriate hair cell phenotypes at all positions along both halves, indicating that positional identity has been established by that development time point. However, separation at E6.5 results in a re-patterning of the distal half of the explant such that the entire tonotopic gradient (based on hair cell density and expression of Calbindin) is represented along the shortened BP ( Fig. 1h,i and Supplementary Fig. 1 ). In contrast, while hair cells do develop in proximal half explants, no evidence of tonotopic identity is present ( Fig. 1h,i , Supplementary Fig. 1 ). These results suggest that tonotopic identity along the BP is determined before E7 and that a potential signalling centre is located at its distal tip. Graded expression of mRNAs along the BP tonotopic axis To identify potential candidate molecules that could be instructive for tonotopic identity, differential expression of mRNAs along the tonotopic axis of the developing BP was analysed using both Affymetrix microarrays and RNA-seq ( Supplementary Data 1 and 2 ). Briefly, based on the results of the experiments described above, E6.5 BPs were dissected and separated into proximal and distal halves (microarray) or proximal, middle and distal thirds (RNA-seq) before isolation of mRNA. Microarray data were analysed to identify transcripts that were expressed at levels at least twofold higher in proximal versus distal halves and gene ontology analysis was used to identify relevant developmental pathways with differential activity in different halves of the BP. The pathways represented by the highest number of differentially expressed transcripts were those associated with cytoskeleton remodelling, in particular members of the transforming growth factor (TGF)-β/Bmp signalling pathway. We were interested in the high number of differentially expressed transcripts related to TGF signalling ( Fig. 2a ), as this pathway has been shown to regulate developmental patterning in a number of tissues and several members have been suggested to act as morphogens [21] . Of the genes known to act within this pathway, transcripts for Bmp7 showed the highest fold difference between proximal and distal regions ( Fig. 2 and Supplementary Figs 9, 10) (2.9-fold difference in transcript expression measured by Affymetrix array and a twofold difference in transcript expression as measured by RNA-seq; Fig. 2a , Supplementary Fig. 2 ). Consistent with this observation, two Bmp-immediate response genes, Id1 and Id3 , were also enriched in the distal half of the BP ( Supplementary Figs 9, 10 and data 3 ). In addition, transcripts for several naturally occurring antagonists of Bmp were found to be expressed at higher levels in the proximal region of the BP ( Fig. 2a ). Finally, the higher level of expression of transcripts for Bmp7 in the distal region of the BP was also consistent with the location of a signalling centre at the distal tip, as was suggested from the results of the separation experiments. 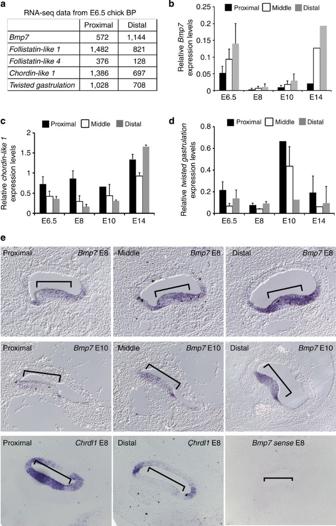Figure 2:Bmp7is expressed in a gradient along the tonotopic axis of the BP. (a) Differential expression of members of the Bmp signalling pathway in proximal and distal regions of the BP at E6.5. Data are presented as the average PMMR (sequences per million mapped reads) forBmp7,Follistatin-like 1 & 4,chordin-like 1andTwisted gastrulation(see text for further details). All experiments were run in triplicate (n=3). (b) Expression ofBmp7in BP tissue from the indicated regions and time points based on quantitative real-time PCR (qPCR) data. An increasing proximal-to-distal gradient is present at all four time points. (c) qPCR data forChordin-like 1(Chdl1) indicates the presence of a counter (decreasing proximal-to-distal) gradient toBmp7between E6.5 and E10. (d)Twisted gastrulation, which acts to enhance the effects ofChordin-like 1, is also present in a decreasing proximal-to-distal gradient between E6.5 and E10. Forb–d, data are mean±s.e.m. andn=4 for each developmental age and position along the BP. (e)In situ hybridizationforBmp7at E8 (top), E10 (middle) andChdl1(bottom) in cross-sections through the BP at the indicated locations. BothBmp7andChdl1are expressed in the developing sensory epithelium of the BP (brackets) and gradients of expression are evident. A sense control forBmp7(bottom right) was negative. Figure 2: Bmp7 is expressed in a gradient along the tonotopic axis of the BP. ( a ) Differential expression of members of the Bmp signalling pathway in proximal and distal regions of the BP at E6.5. Data are presented as the average PMMR (sequences per million mapped reads) for Bmp7 , Follistatin-like 1 & 4 , chordin-like 1 and Twisted gastrulation (see text for further details). All experiments were run in triplicate ( n =3). ( b ) Expression of Bmp7 in BP tissue from the indicated regions and time points based on quantitative real-time PCR (qPCR) data. An increasing proximal-to-distal gradient is present at all four time points. ( c ) qPCR data for Chordin-like 1 ( Chdl1 ) indicates the presence of a counter (decreasing proximal-to-distal) gradient to Bmp7 between E6.5 and E10. ( d ) Twisted gastrulation , which acts to enhance the effects of Chordin-like 1 , is also present in a decreasing proximal-to-distal gradient between E6.5 and E10. For b – d , data are mean±s.e.m. and n =4 for each developmental age and position along the BP. ( e ) In situ hybridization for Bmp7 at E8 (top), E10 (middle) and Chdl1 (bottom) in cross-sections through the BP at the indicated locations. Both Bmp7 and Chdl1 are expressed in the developing sensory epithelium of the BP (brackets) and gradients of expression are evident. A sense control for Bmp7 (bottom right) was negative. Full size image To confirm these results, quantitative real-time PCR (qPCR) was carried out on proximal, middle and distal samples from BPs collected at three different developmental time points. Results confirmed the expression of a dynamic but persistent proximal-to-distal gradient of Bmp7 even in post-hatch BPs ( Fig. 2b ). Interestingly, a marked decrease in overall levels of Bmp7 expression occurs between E8 and E10, although levels of Bmp7 recover to E6.5 levels by post-hatch ages. Similarly, qPCR also confirmed proximal-to-distal gradients of Chordin-like 1 ( Chrdl1 ) and Twisted gastrulation between E6.5 and E10. However, unlike Bmp7 , these gradients do not persist into post-hatch ages ( Fig. 2c,d ). Finally, because the tissue used for microarray, RNA-seq and qPCR contained both sensory epithelium and underlying mesenchymal cells, in situ hybridization was performed to localize Bmp7 and Chrdl1 at E7. Cross-sections indicate that Bmp7 is expressed within the epithelium of the BP with increasing intensity at more distal positions at both E8 and E10 ( Fig. 2e and Supplementary Fig. 2 ). Chrdl1 is also expressed within the epithelium but in a counter-gradient to Bmp7 with more intense expression in more proximal sections ( Fig. 2e ). Bmp7 regulates identity along the tonotopic axis of the BP To investigate a role for the gradient of Bmp7 in the establishment of tonotopy, intact BP explants were established at E6.5 and maintained in control media or media containing 0.4 μg ml −1 Bmp7 for 6 DIV. As described, control BPs developed a normal tonotopic gradient in vitro . In contrast, while distal regions of BPs from Bmp7-treated explants appeared comparable to controls, a significant increase in cell density was present in the more proximal regions of the BP ( Fig. 3a–c ). The increase in proximal cell density was sufficient to completely eliminate the density gradient in these explants (no significant difference between distal and proximal values ( Fig. 3c ). To confirm that the change in cell density was a result of a change in positional identity, additional tonotopic markers were also examined. Average hair cell lumenal surface area in the proximal region of the BP was significantly decreased in Bmp7-treated explants consistent with the acquisition of a more distal identity ( Fig. 3b,d ). As was the case for hair cell density, Bmp7 treatment had no effect on lumenal surface areas of distal hair cells. 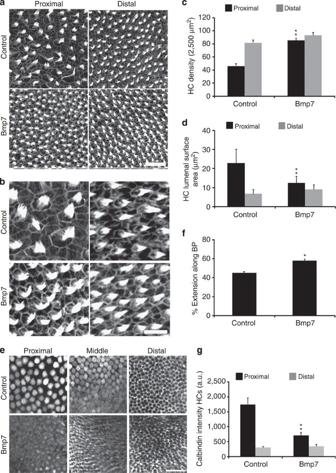Figure 3: Bmp7 specifies positional identity along the tonotopic axis of the BP. (a) Maximumzprojections from the regions indicated BP explant cultures labelled with phalloidin. BPs were maintained for 6 DIV from E6.5 in control media or media supplemented with 0.4 μg ml−1Bmp7. While hair cell density is comparable between the two conditions in the distal region of the BP, a marked increase in density is present in the proximal region of the Bmp7-treated explant. (b) Higher-magnification images from the sample ina. (c) Quantification of changes in hair cell density in the indicated regions in response to Bmp7 treatment. Treatment with Bmp7 causes a significant increase in hair cell density in the proximal region of the BP. As a result, the gradient of hair cell density across the tonotopic axis is abolished. (d) Quantification of mean hair cell lumenal surface area in control and Bmp7-treated cultures in the indicated regions of the BP. Bmp7 treatment induces a significant decrease in proximal hair cells but has no effect on distal hair cells. (e) BP explants established at E6.5, maintained for 6 DIV and then labelled with anti-Calbindin. In the Bmp7-treated explant, Calbindin expression in proximal hair cells appears comparable to expression in hair cells located in the middle region in controls. Similarly, hair cells located in the middle region in Bmp7-treated explants appear to be negative for Calbindin, a phenotype that is restricted to the distal region in control BPs. (f) Quantification of the extension of the distal calbindin phenotype (hair cells negative for Calbindin) along the tonotopic axis from the distal tip in control and Bmp7-treated explants. Bmp7 causes a significant increase in the distal extension of this phenotype. (g) Quantification of mean Calbindin intensity in hair cells from proximal and distal regions of the BP in control and Bmp7-treated explants. Bmp7 treatment causes a significant decrease in Calbindin expression in proximal hair cells. Data are presented as mean±s.e.m. *P<0.02, **P<0.01, based on Student’st-test + Bonferroni correction. Scale bars:a, 100 μm;b, 10 μm;e, 100 μm. For controlsn=14 and for Bmp7-treatedn=8. Figure 3: Bmp7 specifies positional identity along the tonotopic axis of the BP. ( a ) Maximum z projections from the regions indicated BP explant cultures labelled with phalloidin. BPs were maintained for 6 DIV from E6.5 in control media or media supplemented with 0.4 μg ml −1 Bmp7. While hair cell density is comparable between the two conditions in the distal region of the BP, a marked increase in density is present in the proximal region of the Bmp7-treated explant. ( b ) Higher-magnification images from the sample in a . ( c ) Quantification of changes in hair cell density in the indicated regions in response to Bmp7 treatment. Treatment with Bmp7 causes a significant increase in hair cell density in the proximal region of the BP. As a result, the gradient of hair cell density across the tonotopic axis is abolished. ( d ) Quantification of mean hair cell lumenal surface area in control and Bmp7-treated cultures in the indicated regions of the BP. Bmp7 treatment induces a significant decrease in proximal hair cells but has no effect on distal hair cells. ( e ) BP explants established at E6.5, maintained for 6 DIV and then labelled with anti-Calbindin. In the Bmp7-treated explant, Calbindin expression in proximal hair cells appears comparable to expression in hair cells located in the middle region in controls. Similarly, hair cells located in the middle region in Bmp7-treated explants appear to be negative for Calbindin, a phenotype that is restricted to the distal region in control BPs. ( f ) Quantification of the extension of the distal calbindin phenotype (hair cells negative for Calbindin) along the tonotopic axis from the distal tip in control and Bmp7-treated explants. Bmp7 causes a significant increase in the distal extension of this phenotype. ( g ) Quantification of mean Calbindin intensity in hair cells from proximal and distal regions of the BP in control and Bmp7-treated explants. Bmp7 treatment causes a significant decrease in Calbindin expression in proximal hair cells. Data are presented as mean±s.e.m. * P <0.02, ** P <0.01, based on Student’s t -test + Bonferroni correction. Scale bars: a , 100 μm; b , 10 μm; e , 100 μm. For controls n =14 and for Bmp7-treated n =8. Full size image Changes in the gradient of Calbindin expression in hair cells in response to Bmp7 were also consistent with changes in tonotopic identity ( Fig. 3f ). In particular, Calbindin-negative hair cells, which are normally restricted to the distal third of the BP were observed along the distal half of the BP ( Fig. 3f ). Quantification of this effect indicated a significant increase in the extent of Calbindin-negative hair cells towards the proximal end ( Fig. 3f ). The expression of Calbindin in BP supporting cells also extended into the middle region in response to Bmp7 treatment ( Fig. 3e ), suggesting a change in supporting cell positional identity as well. To further quantify the change in Calbindin expression, the intensity of Calbindin-mediated fluorescence in hair cells was assayed in proximal and distal regions of the BP ( Fig. 3g ). While not as profound as the changes observed for hair cell density or lumenal surface area, a significant decrease in Calbindin expression was observed in proximal hair cells in response to Bmp7 treatment. Finally, changes in stereociliary bundle length and size in response to Bmp7 were also examined. Bmp7 treatment induced a significant increase in the length of proximal stereocilia but had no significant effect on distal stereocilia length ( Fig. 4a,b ). Treatment with Bmp7 also significantly reduced the number of stereocilia per bundle on proximal hair cells ( Fig. 4a,c ). Overall, treatment with Bmp7 results in significant changes in multiple tonotopic characteristics all of which are consistent with induction of a more distal phenotype in the proximal end of the BP. To confirm that the effects of Bmp7 do not represent inhibition of a specific cellular pathway phenotype, such as ciliagenesis, BP explants were established at E14 and maintained for 4DIV in the presence of Bmp7. Results indicated no changes between control and Bmp7-treated explants ( Supplementary Fig. 3 ). 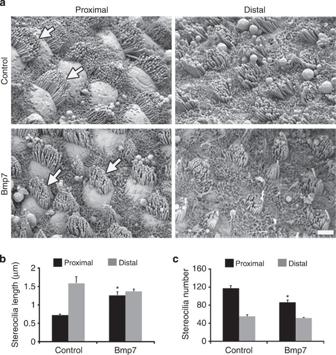Figure 4: Bmp7 treatment alters stereociliary bundle morphology in the proximal region of the BP. (a) SEM images of hair cells in the indicated regions of the BP following following 6 DIV in control or Bmp7-media. Bmp7 treatment leads to notably smaller bundles in the proximal region of the BP. (b) Quantification of the mean length of the longest stereocilia within bundles located on proximal (black bars) or distal (grey bars) hair cells. Bmp7 induces a significant increase in the mean length of the longest stereocilia of proximal hair cells. (c) Quantification of mean number of stereocilia per hair bundle in proximal (black bars) and distal (grey bars) hair cells under the specified conditions. Bmp7 treatment induces a significant decrease in the number of stereocilia per bundle in proximal hair cells. Bmp7-induced changes in hair cell stereocilia are indicated (white arrows). Data are presented as mean±s.e.m. *Pvalue<0.05 based on Student’st-test. For controlsn=4 and for bmp7-treatedn=4. Figure 4: Bmp7 treatment alters stereociliary bundle morphology in the proximal region of the BP. ( a ) SEM images of hair cells in the indicated regions of the BP following following 6 DIV in control or Bmp7-media. Bmp7 treatment leads to notably smaller bundles in the proximal region of the BP. ( b ) Quantification of the mean length of the longest stereocilia within bundles located on proximal (black bars) or distal (grey bars) hair cells. Bmp7 induces a significant increase in the mean length of the longest stereocilia of proximal hair cells. ( c ) Quantification of mean number of stereocilia per hair bundle in proximal (black bars) and distal (grey bars) hair cells under the specified conditions. Bmp7 treatment induces a significant decrease in the number of stereocilia per bundle in proximal hair cells. Bmp7-induced changes in hair cell stereocilia are indicated (white arrows). Data are presented as mean±s.e.m. * P value<0.05 based on Student’s t -test. For controls n =4 and for bmp7-treated n =4. Full size image Inhibition of Bmp7-signalling induces proximal phenotypes To determine whether inhibition of Bmp7 signalling leads to phenotypic changes consistent with induction of a more proximal phenotype, explants were treated with two different Bmp antagonists, Noggin and Chrdl1. Transcripts for Noggin were not detected in the embryonic BP based on Affymterix data and were detected only at very low levels in the RNA-seq results. However, Noggin is a well-characterized and potent antagonist of Bmp and was therefore used as a generic antagonist of Bmp signalling. In contrast, transcripts for Chrdl1 are expressed in a proximal-to-distal gradient along the BP at E6.5 ( Fig. 2 ). Explants treated with either 0.4 μg ml −1 Chrdl1 or 2.5 μg ml −1 Noggin demonstrated changes to the distal end of the BP that are consistent with the induction of a more proximal phenotype ( Fig. 5a ). In particular, significant changes in the distal region of the BP were observed for hair cell density (decreased) and lumenal surface (increased) ( Fig. 5b ). No changes were observed in the proximal region of the BP. The initially tested concentrations of both Bmp7 and Chdl1 were relatively high because of the potential for limited penetration in an explant culture comprising both epithelial and mesenchymal cells. Therefore, to determine the effective concentrations for both Bmp7 and Chrdl1, dose responses were examined for cell density and lumenal surface areas ( Supplementary Fig. 4 ). Results indicated fairly narrow sensitivity ranges for both with 0.25 μg ml −1 of either protein eliciting no effect while a concentration of 0.325 μg ml −1 or above elicited maximal effects ( Supplementary Fig. 4 ). These results suggest that the counter-gradients of both Bmp7 and Chrdl1 may play important roles in the specification of tonotopic identity. 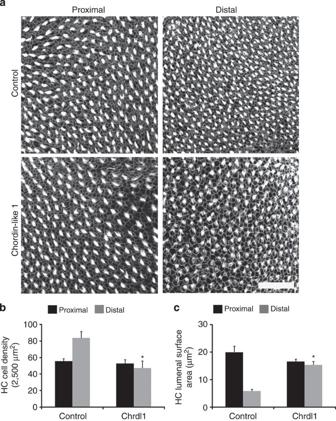Figure 5: Treatment with Chordin-like 1 induces proximal phentoypes in the BP. (a) Maximalzprojections of the surface of BP explants labelled with phalloidin after 6 DIV in control media or media containing 0.4 μg ml−1of Chrdl1. Note the decreased density of hair cells in the distal region in response to treatment with Chrdl1. (b) Hair cell density measured in a 2,500 μm2region at the proximal (black bars) and distal (grey bars) end of the chick BP following 6 DIV in control media, or Chrdl1-media. A significant decrease in hair cell density is observed in the distal region. (c) Lumenal surface areas for hair cells at the proximal (black bars) and distal (grey bars) ends of BP explants following 6 DIV in control media of media containing Chrdl1. Chrdl1 caused a significant increase in lumenal surface area in distal hair cells. Data are presented as mean±s.e.m. *P<0.05 based on Student’st-test. Scale bar, 50 μm. For controlsn=8, and for Chrdl1-treated culturesn=5. Scale bar ina, 100 μm. Figure 5: Treatment with Chordin-like 1 induces proximal phentoypes in the BP. ( a ) Maximal z projections of the surface of BP explants labelled with phalloidin after 6 DIV in control media or media containing 0.4 μg ml −1 of Chrdl1. Note the decreased density of hair cells in the distal region in response to treatment with Chrdl1. ( b ) Hair cell density measured in a 2,500 μm 2 region at the proximal (black bars) and distal (grey bars) end of the chick BP following 6 DIV in control media, or Chrdl1-media. A significant decrease in hair cell density is observed in the distal region. ( c ) Lumenal surface areas for hair cells at the proximal (black bars) and distal (grey bars) ends of BP explants following 6 DIV in control media of media containing Chrdl1. Chrdl1 caused a significant increase in lumenal surface area in distal hair cells. Data are presented as mean±s.e.m. * P <0.05 based on Student’s t -test. Scale bar, 50 μm. For controls n =8, and for Chrdl1-treated cultures n =5. Scale bar in a , 100 μm. Full size image A localized source of Bmp7 alters hair cells density In the experiments described above, the concentration of Bmp7 was altered throughout the entire BP, suggesting the possibility that the phenotypic changes observed could be a result of secondary or tertiary responses to altered Bmp7 signalling. To confirm that Bmp7 acts directly within the BP to alter positional phenotypes, beads soaked in Bmp7 or vehicle (BSA) were placed at the proximal end of E6.5 BP explants. Previous studies have demonstrated that Bmp7 protein released from beads diffuses over an average range of 10–20 cells within a given tissue [22] . By comparison with control beads, a significant increase in hair cell density and a significant decrease in lumenal hair cell surface area were observed within a 2,500 μm 2 area located immediately adjacent to Bmp7-soaked beads ( Supplementary Fig. 5 ). These results are consistent with a direct effect of an increased concentration of Bmp7 on hair cell phenotypes within the BP. In ovo expression of Bmp7 alters hair cell morphologies To confirm that changing the Bmp7 gradient is sufficient to alter positional identity along the BP, we used in ovo electroporation of the otocyst at E2.5 to drive expression of an RCAS-AcGFP-IRES-Bmp7 construct in the inner ear. Visualization of expression of AcGFP confirmed expression of either the RCAS-AcGFP-IRES-Bmp7 or RCAS-AcGFP control vector within the BP at E14 with a bias towards expression in the supporting cells ( Fig. 6a ), as has been reported for previous studies using in ovo electroporation [23] , [24] , [25] . The overall number of viral-expressing cells varied between experiments; however, viral expression was consistently observed in the proximal region of the BP. Analysis of BPs electroporated with the control vector showed development of a normal tonotopic gradient including changes in hair cell density, lumenal surface area and bundle shape and size ( Fig. 6a,b ). In contrast, expression of the Bmp7 construct resulted in significant changes in proximal morphologies that were comparable with the effects of Bmp7 treatment in vitro ( Fig. 6b ). In particular, electroporation of the Bmp7 construct induced a significant increase in hair cell density ( Fig. 6c ), and a significant decrease in lumenal surface area ( Fig. 6d ). In addition, while the precise length and number of stereocilia could not be determined by SEM analysis (because of the limited sample size, n =4 for control and n =7 for Bmp7 ), the overall area of the bundles located on proximal hair cells decreased significantly ( Fig. 6e ), suggesting a reduction in the number of stereocilia per bundle. Moreover, the morphology of these bundles was consistent with distal rather than proximal hair cells ( Fig. 6b ). No significant changes were observed in hair cells located at the distal ends of BPs transfected with RCAS-AcGFP-IRES-Bmp7 ( Fig. 6 ). For quantification of bundle area please refer to the Methods section. 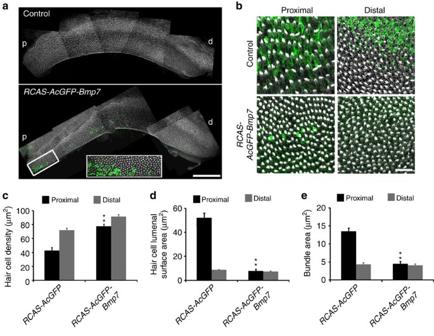Figure 6: Over-expression of Bmp7in ovoalters positional identity along the tonotopic axis. (a) Low-magnification montage images of E14 BPs electroporated with eitherRCAS-AcGFP(control) orRCAS-AcGFP-Bmp7at E2.5. Images show BPs labelled with phalloidin (white) to visualize stereociliary bundles and anti-GFP (green) to visualize infected cells. Electroporation does not alter the normal morphology of the developing BP. (b) High-magnification images of the indicated regions of the BP from control (top) andRCAS-AcGFP-Bmp7(bottom) samples labelled as ina. Expression ofBmp7in the proximal region of the BP induces a marked increase in hair cell density and decrease in lumenal surface area. (c) Quantification of changes in mean hair cell density in proximal (black bars) and distal (grey bars) regions of the BP following electroporation withRCAS-ACFGP(control) orRCAS-AcGFP-Bmp7. Proximal hair cell density is significantly increased in the presence ofBmp7. (d) Quantification of mean hair cell lumenal surface area following electroporation. Expression ofBmp7induces a significant decrease in proximal hair cell surface areas. (e) Mean stereociliary bundle area for hair cells located in proximal (black bars) or distal (grey bars) regions of the BP following electroporation with eitherRCAS-AcGFPorRCAS-AcGFP-Bmp7.Bmp7induces significantly decreased bundle area in proximal hair cells. Data are mean ±s.e.m. **P<0.05 based on Student’st-test. Scale bars:a, 200 μm;b, 50 μm. For controlsn=4 and for Bmp7n=7. Figure 6: Over-expression of Bmp7 in ovo alters positional identity along the tonotopic axis. ( a ) Low-magnification montage images of E14 BPs electroporated with either RCAS-AcGFP (control) or RCAS-AcGFP-Bmp7 at E2.5. Images show BPs labelled with phalloidin (white) to visualize stereociliary bundles and anti-GFP (green) to visualize infected cells. Electroporation does not alter the normal morphology of the developing BP. ( b ) High-magnification images of the indicated regions of the BP from control (top) and RCAS-AcGFP-Bmp7 (bottom) samples labelled as in a . Expression of Bmp7 in the proximal region of the BP induces a marked increase in hair cell density and decrease in lumenal surface area. ( c ) Quantification of changes in mean hair cell density in proximal (black bars) and distal (grey bars) regions of the BP following electroporation with RCAS-ACFGP (control) or RCAS-AcGFP-Bmp7 . Proximal hair cell density is significantly increased in the presence of Bmp7 . ( d ) Quantification of mean hair cell lumenal surface area following electroporation. Expression of Bmp7 induces a significant decrease in proximal hair cell surface areas. ( e ) Mean stereociliary bundle area for hair cells located in proximal (black bars) or distal (grey bars) regions of the BP following electroporation with either RCAS-AcGFP or RCAS-AcGFP-Bmp7.Bmp7 induces significantly decreased bundle area in proximal hair cells. Data are mean ±s.e.m. ** P <0.05 based on Student’s t -test. Scale bars: a , 200 μm; b , 50 μm. For controls n =4 and for Bmp7 n =7. Full size image Bmp7 regulates its own expression within the BP To examine the nature of the regulation of Bmp7 expression levels within the BP, changes in expression of Bmp7 mRNA were examined in response to treatment with Bmp7, Noggin or Chrdl1. Exposure to 0.4 μg ml −1 Bmp7 caused a decrease in Bmp7 expression in both proximal and distal regions of the BP although the distal-to-proximal gradient was preserved ( Supplementary Fig. 6 ), indicating that Bmp7 acts as a negative regulator of its own expression. In contrast, treatment with Noggin (2.5 μg ml −1 ) or Chrdl1 (0.4 μg ml −1 ) essentially eliminated expression of Bmp7 along the length of the BP ( Supplementary Fig. 6 ), indicating that some level of Bmp7 signalling is required to maintain its own expression. Bmp7 regulates cell density through a non-mitotic pathway Bmps have been linked with cellular proliferation in other developing systems [26] . To determine whether the increased density in the proximal regions of Bmp7-treated explants was a result of increased proliferation, the mitotic tracer BrdU was added to the culture media along with Bmp7 protein for 6 DIV. Results indicated no increase in BrdU labelling ( Supplementary Fig. 7 ), indicating that Bmp7 influences cell fate rather than proliferation. Bmp7 regulates tonotopy through a non-canonical pathway Bmp7 is known to activate both canonical (Smad) and non-canonical (Tak1/Mapk) signalling pathways. To determine which Bmp pathway acts to regulate tonotopic identity, activation of canonical and non-canonical pathways within the BP was examined following Bmp7 treatment. First, explants were established as described and maintained in the presence of either Bmp4 or Bmp5, both of which strongly activate the canonical Bmp/Smad signalling pathway. In comparison to treatment with Bmp7, incubation of BP explants with either Bmp4 or Bmp5 protein had no significant effect on tonotopic morphometrics in the proximal region of the BP ( Supplementary Fig. 8a,b ). Similarly, no changes were observed in the levels of phospho-Smad 1, pSmad 5 or pSmad 8 (pSmad 1/5/8) in response to treatment with Bmp7 ( Supplementary Fig. 8c ). These results suggest that the effects of Bmp7 are unlikely to be mediated through activation of the canonical Bmp/Smad pathway. Bmp7 is also known to signal through the Map-kinase pathway, in particular by activatingTak1. To determine whether Tak1 activation plays a role in regulation of tonotopic identity, explants were established at E6.5 and maintained for 6 DIV in the presence of the Tak1 inhibitor (5 Z )-7-oxozeaenol. In addition, the downstream targets of Tak1, Jnk and p38 were blocked using the p-Jnk inhibitor SP600125 or the p38 Map-kinase inhibitor SB202190. In contrast with Bmp7 treatment, which causes more distal-like hair cell phenotypes in the proximal BP, inhibition of Tak1, Jnk or p38 resulted in proximal hair cells developing more distal phenotypes. This was characterized by a significant reduction in hair cell density and size of lumenal surface areas in the proximal region of the BP ( Fig. 7a ). To determine whether the Tak1/Jnk/p38 pathway acts in the same pathway as Bmp7, explants were treated with both Bmp7 and one of the three Mapk kinase inhibitors. The presence of any one of the Mapk inhibitors rescued tonotopic development when combined with Bmp7 treatment ( Fig. 7a–d ). These results are consistent with Bmp7 acting through the Tak1/Jnk/p38signaling pathway to regulate tonotopic identity. Finally, activation of Tak1 in response to Bmp7 was confirmed by assaying for changes in levels of phospho-Tak1 following Bmp7 treatment ( Fig. 7e ). E6.5 BPs treated with Bmp7 showed a rapid increase in levels of phospho-Tak1, demonstrating a direct effect of Bmp7 signalling on Tak1 activation. 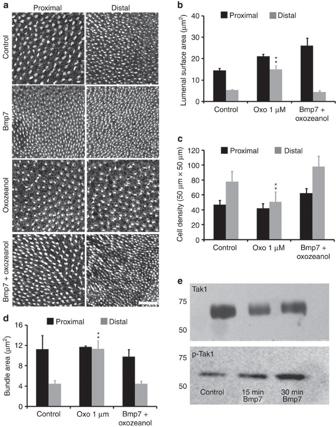Figure 7: Bmp7 modulates positional identity through activation of the Tak1 pathway. (a) Maximumzprojections of phalloidin-labelled BP cultures illustrating hair cell density at the proximal and distal ends of BP explants after 6 DIV under the indicated conditions (see text for details). Inhibition of Tak1 (oxozeanol) induces decreased hair cell density in the distal region of the BP, consistent with a more proximal phenotype. This phenotype contrasts with the effects of Bmp7 and is comparable to the effects of treatment with Chrdl1 (Fig. 4). In contrast, explants treated with both Bmp7 and oxozeanol appear comparable to control. (b) Quantification of mean hair cell density in BPs treated with oxozeanol alone or oxozeanol and Bmp7. Oxozeanol treatment leads to a significant decrease in distal density and elimination of the density gradient. In contrast, treatment with Oxozeanol and Bmp7 has no effect on the density gradient. (c,d). Data show quantification or hair cell lumenal surface area and bundle volume for the same conditions as inb. For both, Oxozeanol treatment induces changes consistent with distalization of the BP while treatment with Oxozeanol and Bmp7 has no effect on tonotopic patterning. All data are presented as mean±s.e.m. Stars indicate aPvalue <0.05, Student’st-test. Controlsn=14, oxozeanoln=5, oxo+Bmp7n=8. (e) Western blot for total (upper) and phosphorylated (lower) Tak1 in E8 BPs in response to treatment with Bmp7. A rapid increase in levels of p-Tak1 is observed following Bmp7 treatment. Scale bar ina, 100 μm. Figure 7: Bmp7 modulates positional identity through activation of the Tak1 pathway. ( a ) Maximum z projections of phalloidin-labelled BP cultures illustrating hair cell density at the proximal and distal ends of BP explants after 6 DIV under the indicated conditions (see text for details). Inhibition of Tak1 (oxozeanol) induces decreased hair cell density in the distal region of the BP, consistent with a more proximal phenotype. This phenotype contrasts with the effects of Bmp7 and is comparable to the effects of treatment with Chrdl1 ( Fig. 4 ). In contrast, explants treated with both Bmp7 and oxozeanol appear comparable to control. ( b ) Quantification of mean hair cell density in BPs treated with oxozeanol alone or oxozeanol and Bmp7. Oxozeanol treatment leads to a significant decrease in distal density and elimination of the density gradient. In contrast, treatment with Oxozeanol and Bmp7 has no effect on the density gradient. ( c , d ). Data show quantification or hair cell lumenal surface area and bundle volume for the same conditions as in b . For both, Oxozeanol treatment induces changes consistent with distalization of the BP while treatment with Oxozeanol and Bmp7 has no effect on tonotopic patterning. All data are presented as mean±s.e.m. Stars indicate a P value <0.05, Student’s t -test. Controls n =14, oxozeanol n =5, oxo+Bmp7 n =8. ( e ) Western blot for total (upper) and phosphorylated (lower) Tak1 in E8 BPs in response to treatment with Bmp7. A rapid increase in levels of p-Tak1 is observed following Bmp7 treatment. Scale bar in a , 100 μm. Full size image The auditory environment comprises myriad complex sounds from subtle wing beats and footfalls to elaborate bird songs and concertos. In order to process and appreciate the complexity of these signals, the auditory systems of many vertebrates reduce these sounds to their component frequencies. Primary auditory sensors spatially separate individual frequencies to create a tonotopic map that is maintained at multiple levels of the auditory system [1] , [10] , [27] . Within these sensors, spectral separation is achieved through changes in a combination of physical, anatomical and physiological characteristics that result in a graded change in maximal frequency sensitivity along the tonotopic axis. In order to achieve this gradient in sensitivity, developing progenitor cells arrayed along the nascent auditory sensor must determine their relative position along the axis. Similar patterning events have been shown to be required for the formation of other structures with graded morphologies such as the three primary body axes, the neural tube and the hind- and forelimb [28] , [29] , [30] , [31] . In many of these cases, gradients of one or more morphogens act to regulate cell fate and morphology along a specific axis [31] , [32] . The results presented here show that a gradient of Bmp7 activity plays a key role in determining positional identity along the tontopic axis of the chick BP. Bmp signalling gradients play similar roles in other patterned structures, most notably in the formation of the dorsoventral axis in vertebrates and imaginal disks in Drosophila [30] , [33] , [34] . In these systems, and others, a largely conserved signalling cassette that includes Bmps, secreted antagonists such as Noggin, Chordin or Chordin-like 1, membrane antagonists such as Bambi and metalloproteases such asTolloid, is expressed across the patterning axis [35] , [36] , [37] , [38] . While not fully validated in this work, tonotopic gradients for Bambi , Tolloid-like1 and ADMP-like were observed within the E6 BP ( Supplementary Data 1 ). Therefore, it seems likely that determination of tonotopic identity along the BP utilizes multiple components of this conserved signalling network. The involvement of the Bmp patterning cassette provides an explanation for the observation of at least a partial re-patterning of the full tonotopic axis in isolated distal halves of the BP. Work from De Robertis and colleagues and others [30] , [39] , [40] have demonstrated the existence of multiple feedback loops that communicate between dorsal and ventral signalling centres to provide self-regulation along a specific axis. Loss of the proximal chordin-like signalling centre, as would occur following separation into distal and proximal halves, could for example be compensated for by an increased expression of the Bmp antagonist Bambi in the distal half, leading to re-establishment of a gradient of Bmp signalling. Our data are also consistent with the requirement for tonotopic patterning to be scalable across species with different body mass, head size and BP length [41] . Conversely, there is no compensation for the loss of the distal Bmp signalling centre. In contrast with the apparent conservation of the use of the Bmp/Chordin patterning cassette, our results suggest that regulation of positional identity along the BP is not mediated through the canonical Bmp/Smad pathway. Instead, we show that Bmp7 functions through activation of the Tak1/Mapk pathway. While this is considered to be a non-canonical Bmp pathway, Tak1 is known to be a downstream effector of TGFβ/Bmp signalling [42] and acts throughout vertebrate development [43] . In particular, Tak1 has a role in vascular formation and angiogenesis, where it regulates both expression of angiogenic genes and cell migration [44] , [45] , and in the developing kidney where it is essential for maintenance and regulation of cell number within the nephron progenitor pool [26] . While this study marks the first demonstration of a role for Tak1 in development of the auditory system, a recent report demonstrated broad expression of Tak1 in the mouse otocyst and cochlea [46] . A crucial next step will be to determine the Tak1 targets that mediate specific aspects of hair cell positional identity. The dynamic nature of the Bmp7 gradient has intriguing implications for both BP development and regeneration. While a distal-to-proximal gradient was observed both during embryonic development of the BP and in post-hatch chicks, the relative levels of Bmp7 changed. At E8 and E10, Bmp7 mRNA expression levels decreased significantly by comparison with the levels present at E6.5, but by P14 levels had returned to, or even exceeded, those observed at E6.5. The basis for the decrease in Bmp7 between E8 and E10 is unclear but the result of this decrease may be the relief of an active suppression of Raldh3 leading to the formation of a distal-to-proximal gradient of retinoic acid (RA) at E10 (Thiede et al ., co-submission). Modulation of the RA gradient alters stereocilia number and length in patterns consistent with changes in positional identity (Thiede et al ., co-submission). The timing of this change correlates with previous descriptive work indicating specification of cell fates between E6.5 and E9 followed by development of stereocilia bundles beginning around E10 (ref. 4 ). The data presented here and in Thiede et al . suggest that the gradient of Bmp7 at E6.5 regulates the specification of overall positional identity, while the formation of an RA gradient at E10 acts more specifically to regulate bundle morphology. In contrast with some developmental patterning events in which a morphogen is localized to a point source at one end of a graded structure, such as the localization of Sonic hedgehog to the ventral floor plate cells of the neural tube [47] , gradients of transcripts for Bmp7 and several Bmp antagonists are present along the length of the BP as early as E6.5. These results suggest that even though positional identity is not yet fully determined at this time point, as demonstrated by the separation experiments, progenitor cells along the tonotopic axis already have information regarding their location. The cues and/or signalling pathways acting upstream of Bmp7 are unknown. In the chick, since the developing BP extends primarily along the primary medio-lateral body axis, it is possible that cues originating from central structures such as the neural tube or notochord could establish initial positional identity along the developing BP. Alternatively, cues could arise from the otocyst itself either in the form of diffusible factors or as a result of temporal or migratory cues [48] . Further experiments are clearly required to address these possibilities. Previous work has demonstrated that regenerated hair cells develop location-appropriate morphological and physiological characteristics, suggesting regenerating hair cells can determine their position along the tonotopic axis [8] , [49] . The finding that a distal-to-proximal gradient of Bmp7 is present in post-hatch BPs suggests a possible instructive role during regeneration. If relative expression of Bmp7 acts as a place code, then expression in the location-specific supporting cells that give rise to regenerated hair cells could provide positional information. Alternatively, if regenerated hair cells arise without a specified positional identity, then the presence of the Bmp7 gradient in cells surrounding new hair cells could provide positional information to those cells as they mature. Embryo care and procedures Fertilized White Leghorn chicken ( Gallus gallus Domesticus ) eggs (B & E eggs, PA) were incubated at 37.5 °C in an automatic rocking incubator (Brinsea) until use at specific developmental stages between E6 and E14. Embryos were removed from their eggs, staged according to Hamburger and Hamilton [50] and subsequently decapitated. All embryos were terminated before hatching at E21. All procedures were approved by the Animal Care and Use Committees at the NIH or at the University of Virginia. BP culture BPs were isolated from embryos incubated for between 6 (E6.0) and 8 days and maintained in chilled Leibovitz’s L-15 media (GIBCO, Invitrogen). Papillae were dissected as described previously [51] . Isolated BPs were cultured on Matrigel-coated (BD Biosciences, San Jose, CA, USA) Millicell cell culture inserts (Millipore). Cell culture inserts were placed into 35-mm culture dishes containing 1.5 ml of Basal medium Eagle (GIBCO, Invitrogen) supplemented with 5 mM HEPES buffer. Papillae were maintained in Basal medium Eagle plus vehicle (control media) for up to 6 DIV until the equivalent of embryonic day 12 (E12). For separation experiments, BPs were dissected as described on specific days and then separated at the mid-point of the BP to create distal and proximal halves that were then cultured in separate dishes. Separated explants were maintained for 6 DIV. For separation experiments at specific ages, a minimum of four samples were analysed. The following factors were applied to experimental BPs at specific concentrations described in the text: Bmp7 (R&D systems), Bmp4 (R&D systems), Bmp5 (R&D systems), Noggin (R&D systems), SP600125 (Sigma), SB203580 (Sigma), Fgf3 (R&D systems) or Chordin-like 1 (Chrdl1, R&D systems). At the conclusion of each experiment, cultures were fixed in 4% paraformaldehyde (PFA) for 30 min at room temperature (RT), washed thoroughly three times with 0.1 M phosphate-buffered saline (Invitrogen) and processed for immunohistochemistry. RNA isolation and first-strand cDNA synthesis BP tissue was either dissected immediately following removal from the embryo and divided into proximal and distal halves, or processed following 6 DIV. The lagena and vestibular organs were removed as completely as possible before tissue was processed for RNA isolation. Regardless of condition, total RNA was extracted using the RNAqueous-Microkit (Ambion). First-strand cDNA synthesis was performed using the SuperScriptIII first-strand synthesis kit (Invitrogen) using random priming with 100 ng of template. Affymetrix microarray analysis RNA was extracted from 20 proximal and 20 distal BP samples collected on 3 separate days allowing for triplicate biological replicates of each microarray experiment. RNA was extracted as described previously using the RNAqueous-Microkit (Ambion). Total RNA was further purified on an RNAeasy column (Qiagen) and the RNA quality was checked by an Agilent Bioanalyzer (Agilent Technologies, Palo Alto, CA, USA). Target labelling and hybridization to GeneChips were carried out in the NIDDK Microarray Core facility using the GeneChip Mouse 430_2 Array purchased from Affymetrix. The microarray signals were normalized using the RMA algorithm. The mRNAs expressed at significantly different levels in distal versus proximal BP were selected based on ANOVA analysis by Partek Genomics Suite software (Partek, St Charles, MO, USA). The ANOVA gene lists by P value of 0.05 and absolute value of fold change of 1.5 including up- and downregulated genes were used in the gene ontology analysis by the commercial gene pathway analysis web tool ( http://trials.genego.com/cgi/index.cgi ). Next-gen sequencing using the Illumina platform Polyadenylated RNAs from total RNA were purified by conventional methods (oligo (dT) beads) and the mRNAs were randomly fragmented by heat treatment. First-strand cDNA was carried out using random priming and RT-mediated cDNA synthesis, followed by second-strand cDNA synthesis and end repair. A single A residue was then added to each cDNA end (necessary for Illumina linker ligation) and ligated to the Illumina amplification/sequencing linkers. Using gel purification, we generated a range of cDNA fragments [200 bp (±25 bp)) optimally suited for the Illumina sequencing technology. In brief, mRNA was selected using oligo-dT magnetic beads and fragmented. First-strand cDNA was synthesized using random primers. Second-strand synthesis, end repair, addition of a single Abase and adaptor ligation were then performed. Each RNA-seq library was subsequently sequenced using either the Illumina Genome Analyser IIx or HiSeq2000. RNA-Seq data analyses Sequence data were aligned with the Ensembl Gallus gallus reference genome (WUGSC2.1) using Tophat v1.4.0 (ref. 52 ). Data output. bam files were processed by Partek Genomics Suite v6.6 (Partek Inc., St Louis, MO, USA) to assemble reads into transcripts and estimate their expressions level. A gene model data set combining Ensembl and NCBI annotations was used to generate RPKM (reads per kilobase of exon per million fragments mapped) for both known genes and uncharacterized transcripts. Statistical tests were carried out using one-way analysis of variance (ANOVA). A minimum value of ⩾ 0.5 RPKM, in addition to a fold change of ⩾ 2 was required for consideration of differential expression between distal and proximal regions. Real-time quantitative PCR Real-time PCR was performed using a Step One Plus real-time PCR machine (Applied Biosystems). All reactions were performed using the qPCR core kit for SybrGreen (Applied Biosystems). Real-time PCR on test samples was carried out in triplicate using appropriate forward and reverse primers for Bmp7 (forward: 5′-TGGTCATGAGCTTCGTCAAC-3′; reverse: 5′-CCTCTGGGATTCTGGAGAGA-3′), Chrdl1 (forward: 5′-GTGTGCTCTGTCTCCTGCTC-3′; reverse: 5′-AAGCCCGTAGGGTTCTAGGT-3′) and Twisted Gastrulation (forward: 5′-CAAGCAACAACATCCACGCA-3′; reverse: 5′-GCACTCTGGCCCAATACACT-3′). For TaqMan assays, total RNA was also reverse-transcribed using SuperScriptIII first-strand synthesis kit (Invitrogen). Quantitative real-time PCR was performed on cDNA samples and no template controls using custom-designed fluorogenic TaqMan probes (Integrated DNA Technologies (IDT), Inc.) and brilliant III fast QPCR mastermix (Agilent). Amplification of target genes was detected using the Step One Plus real-time PCR machine (Applied Biosystems). Inter-sample variation was corrected for by normalizing gene expression levels to internal levels of the ‘housekeeping gene’ large ribosomal protein ( RPLPO ) reference (forward: 5′-GTCACATCACAGGGAGCAAT-3′; reverse: 5′-GCTTTGTGTTCACCAAGGAG-3′). In situ hybridization Inner ear tissue was dissected and fixed in 4% PFA overnight at 4 °C. Tissue was subsequently washed for 30 min in 0.1 M PBS before cryoprotection with sucrose (10–30% solutions diluted in 0.1 M PBS+0.02% Tween 20) and OCT. Frozen tissue sections were cut at a thickness of 12 μm. For whole-mount in situ , tissues were fixed in 4% PFA overnight at 4 °C, washed thoroughly in 0.1 M PBS and subsequently dehydrated in methanol (25–100%). Tissue was stored at −20 °C until use. Immediately before the in situ protocol, tissue was rehydrated using a reverse methanol gradient (100–25%). Complimentary digoxigenin-labelled RNA probes for Bmp7 were kindly provided by Doris Wu (NIDCD, NIH). All in situ hybridization reactions were performed as described previously [53] . Generation of in situ probes In situ probes for Chicken Chordin-like 1 ( Chrdl1 , NM_204171.1), Follistatin-like 1 ( Fstl1 , NM_204638.1) and Twised Gastrulation Homolog1 ( Twsg1 , NM_204198.1) were prepared from cDNA, which was cloned by RT–PCR from RNA extracted from E5 chicken embryos, using the following primers: Chrdl1 -788 (forward, 5′-CACCACGGCGAAATGTTTGT-3′; Chrdl1 -1697 (reverse, 5′-GGCTGATCTGAGCTTCTCCC-3′; Fstl1 -76 (forward, 5′-TCTGGAAAACTCTCCCGCTG-3′; Fstl1 -919 (reverse, 5′-TGACCAGGTTGCTGTCTGTG-3′; Twsg1 -489 (forward, 5′-GAACCAGCCACAGCATCAGA-3′; Twsg -1318 (reverse, 5′-ATTTTATCCACGACGGCCCA-3′). Accuracy of all probes was confirmed by sequencing. In situ hybridization was carried out as described above. Immunohistochemistry Following fixation, cultures were permeabilized in 0.1 M PBS containing 0.02% Triton X-100 (SIGMA) for 30 min at RT and subsequently blocked for 1 h with 10% goat or horse serum (Vector Laboratories). Tissue was incubated in primary antibody overnight at 4 °C at the listed dilutions. Antibody staining was visualized using secondary antibodies conjugated to either Alexa488 orAlexa 546 (Invitrogen). Cultures were incubated with all secondary antibodies for 1 h at RT, washed in PBS and then incubated for an additional hour with either Alexa Fluor-conjugated Phalloidin-546 or-633 (Invitrogen) to label filamentous actin. Tissue samples were mounted using either Fluoromount (Invitrogen) or SlowFade (Invitrogen). The following primary antibody was used in this study: mouse monoclonal antibody against Calbindin 28 kDa protein (1:500, Abcam, ab82812). BrdU labelling As described by Burns et al . [54] , BrdU at a concentration of (3 μg ml −1 ) was added to the culture medium at the outset of the experiment and was maintained throughout. At the end of the experiment, BPs were fixed in fresh 4% PFA for 30 min at RT. After fixation, specimens were washed in PBS and then permeabilized and blocked for 1 h at RT in PBS with 0.2% Triton X-100 (PBS-T) and 10% normal goat serum (Invitrogen). Samples were digested with DNAse I (0.5 kunits/μl; Sigma) for 1 h at 37 °C before adding the blocking solution. Samples were then incubated in mouse anti-BrdU (1:50, BD Biosciences) in PBS-T with 2% normal goat serum overnight. Primary antibody labelling was visualized with AlexaFluor-conjugated secondary antibodies (1:200, Invitrogen) in PBS-T. Filamentous actin was then visualized as described above. In ovo electroporation The mouse Bmp7 cDNA sequence was obtained from Open Biosystems and was sub-cloned into the pIRES2-AcGFP1 vector (Clontech) using in-fusion cloning (Clontech). The AcGFP-IRES and AcGFP-IRES-Bmp7 sequences were subsequently excised and ligated into the Cla1 site of the replication competent ASLV ( avian sarcoma-leukosis virus ) long terminal repeat with a splice acceptor, Bryan polymerase, and B envelope (RCASBP (B)) vector [55] to generate either the RCASBP (B)-AcGFP or RCASBP (B)-AcGFP-IRES-Bmp7 constructs. Expression plasmids were then prepared using an endotoxin free purification kit (Machery Nagel). Electroporation of the chick otic cup was performed as described previously by Daudet and Lewis [56] . Embryos were staged according to the Hamburger and Hamilton guide [57] and DNA was electroporated into the otic cup at stage 13 (48–52 h). Following successful electroporation, embryos were developed until embryonic day 14 (E14) at which time tissue was harvested and processed for immunohistochemistry. Bead implantation BPs were dissected and cultured as described. Agarose beads (Affi-Gel Blue gel, Bio-Rad) were incubated for 1 h at RT in either bovine serum albumin (BSA) (SIGMA Aldrich) or BSA with 0.5 μg μl −1 of Bmp7 protein. Treated beads were subsequently placed at the proximal end of the BP using fine forceps. Cultures were then maintained for 6 days after which they were fixed in 4% PFA and processed for immunohistochemistry. Western blot Protein extracts were prepared from E7 BPs treated with Bmp7 for 15 or 30 min at RT. Tissue was treated with RIPA buffer (SIGMA Aldrich) containing protease (Complete mini; Roche) and phosphatase (SIGMA Aldrich) inhibitor tablets at 4 °C. Tissue was left on ice for 2 h with periodic vortexing. Tissue lysates were subsequently denatured at 85 °C for 5 min with NuPAGE LDS sample loading buffer (Invitrogen) and β-mercaptoethanol (SIGMA Aldrich). Proteins were then separated using SDS–PAGE on a 4–12% gradient Bis-Tris gel (Invitrogen) and subsequently transferred to nitrocellulose membranes (Invitrogen) overnight at 4 °C. The primary antibodies and dilutions used were as follows: Rabbit anti-Tak1 (1:1,000, Cell Signaling), Rabbit anti-phospho-Tak1 (1:1,000, Cell Signaling), rabbit anti-Smad 1/5/8 (1:1,000, Cell Signaling), rabbit anti-phospho Smad 1/5/8 (1:1,000, Cell Signaling) and mouse anti-β-Actin (1:5,000, Sigma Aldrich). Horseradish peroxidase-conjugated anti-rabbit (1:1,000) or anti-mouse (1:5,000) IgGs were used as secondary antibodies (GE Healthcare). Specific bands were visualized by chemiluminescence using the SuperSignal West Pico Chemiluminescenct Substrate kit (Thermo Scientific). Image acquisition and analysis Images were acquired along the entire length of the BP and then at higher magnification at proximal, middle and distal regions using a Zeiss 510 or 710 LSM confocal microscope and × 20 Plan Apochromat (NA 0.8) or × 40 Plan-Neofluar (NA 1.3) objectives. Data were analysed offline using image J software. The following metrics were used as indicators of tonotopic location along the papilla: hair cell density [3] , luminal surface area [3] and expression of Calbindin in hair cells [5] . To determine the hair cell density, the stereociliary bundles and lumenal surfaces of hair cells were labelled with phalloidin. Then, the number of hair cells in 50 μm × 50 μm regions of interest (2,500 μm 2 total area) located at the proximal, middle and distal, or just proximal and distal, regions of the BP were determined. Proximal, middle and distal regions were determined based a calculation of the entire length of the BP or explant. In addition counting boxes were located in the mid-region of the BP along the neural to abneural axis in order to avoid any confounding measurements due to radial differences between tall and short hair cells. For each sample, hair cells were counted in four ROIs for each position along the BP. Lumenal surface areas were determined by measuring the circumference of individual hair cells at the level of the cuticular plate in the same ROIs. Calbindin expression in hair cells was determined using three 2,500 μm 2 ROIs one each located in the distal, middle and proximal regions of the BP. Within each ROI, fluorescence intensity at the lumenal surface of all hair cells based on anti-Calbindin labelling was determined using the LSM 710 analysis tools. Detection parameters for the LSM were determined to ensure that all samples were within the dynamic range of the LSM detector and all analyses were made using the same settings. Fluorescence intensity for each hair cell was normalized to compensate for differences in lumenal surface area and then averaged for all the cells within a single ROI. Number of samples for each experiment are noted in the figure legend but a minimum of three independent samples was included for each experiment. For some experiments, bundle area was calculated based on phalloidin-labelling. Using ImageJ analysis software ROIs were drawn around individual hair cell bundles in images oriented such that the view was perpendicular to the lumenal surface. The average bundle area was calculated for all hair cells within an ROI located at specific positions along the tonotopic axis Bundle area was determined because it was not possible to resolve individual stereocilia at these ages based on phalloidin staining alone. Unless stated otherwise, Student’s t- test with Bonferroni correction was used for all statistical analysis. Scanning electron microscopy BP explants were fixed in 3% glutaraldehyde in 0.10 M cacodylate buffer and 2 mM CaCl 2 at pH 7.35. Tissue was subsequently post-fixed in 1% OsO 4 for 2 h at RT, washed in cacodylate buffer and processed by the Osmium–Thiocarbohydrazide–Osmium method [58] . Tissue was then dehydrated using a graded ethanol series, dried at the critical point, mounted on stubs and sputter-coated with gold palladium. Samples were imaged using a JEOL 6400 scanning electron microscope. SEM analysis To characterize the HC bundle morphology, high-magnification SEM images were taken midway between the inferior and superior edges throughout the BP at the apical surfaces of the HCs. Approximately 20 HCs were analysed for each image. Images were taken at random from three neighbouring fields in the proximal and distal BP regions, providing six images per for analysis per explant. HCs from the extreme proximal and distal edges were not imaged as well as those from extreme superior or inferior edges. Determination of stereocilia number Using SEM, stereocilia were counted from proximal and distal BP regions. The mean number of stereocilia was counted from HCs on which the bundle was clearly identifiable. Quantifications were done blindly. Stereocilial number was measured from scanning electron micrographs taken at 3,500 × 6,000 magnification. Using a bird’s eye view of the bundle, stereocilia were counted with Image J software. The number of stereocilia was determined from at least five hair cells counted in three independent regions at proximal and distal ends of the BP. Length measurements SEM images were acquired from proximal and distal BP regions. At least three images from neighbouring fields were taken midway between the superior and inferior edges of the proximal and distal regions. In order to determine bundle height, the height of the tallest stereocilium was measured. Measurements were analysed with Imaris 64 software. Statistical tests were conducted using GraphPad Prism 8.0. This software was used to measure the maximum length of the entire bundle, as it was not always possible to resolve individual stereocilia. We used the average bundle length as an indicator of stereocilial length. Data was analysed using one-way ANOVA with Newman–Keuls post-test (GraphPad Prism). How to cite this article: Mann, Z. F. et al . A gradient of Bmp7 specifies the tonotopic axis in the developing inner ear. Nat. Commun. 5:3839 doi: 10.1038/ncomms4839 (2014).